Single-pixel imaging by means of Fourier spectrum acquisition Single-pixel imaging techniques enable to capture a scene without a direct line of sight to the object, but high-quality imaging has been proven challenging especially in the presence of noisy environmental illumination. Here we present a single-pixel imaging technique that can achieve high-quality images by acquiring their Fourier spectrum. We use phase-shifting sinusoid structured illumination for the spectrum acquisition. Applying inverse Fourier transform to the obtained spectrum yields the desired image. The proposed technique is capable of capturing a scene without a direct view of it. Thus, it enables a feasible placement of detectors, only if the detectors can collect the light signals from the scene. The technique is also a compressive sampling like approach, so it can reconstruct an image from sub-Nyquist measurements. We experimentally obtain clear images by utilizing a detector not placed in direct view of the imaged scene even with noise introduced by environmental illuminations. An optical imaging system generally consists of an illumination source and a light detection unit. For conventional imaging techniques, a scene is illuminated by a uniform light field and detected with a pixelated array of detectors (charge-coupled device camera, complementary metal oxide semiconductor camera, for example) through some lensing optical system. The light collected by a detector can be divided into direct light and indirect light ( Supplementary Fig. 1 ). Direct light is any light that has not been scattered before falling on the detector while indirect light refers to light that has been scattered before falling on the detector. Direct light contributes to an effective signal, while in most cases indirect light contributes to noise. Therefore, it is difficult for the conventional techniques to capture a scene with a small amount of direct light detected (for instance, objects hidden behind scattering media or around a non-specular corner) due to the resulting low signal-to-noise ratio (SNR). The first approach attempted with single-pixel imaging might have been the ‘flying-spot’ camera patented in 1884 by Paul Nipkow who proposed the use of a perforated disk (also known as a Nipkow disk) to modulate a light source for scanning light spots across a scene [1] . Although several improved flying-spot cameras were proposed later, this approach has been out of favour because of the low SNR. In recent years, a number of novel single-pixel imaging techniques have been presented. The single-pixel imaging techniques are often referred to ghost imaging (GI). Conventional GI [2] exploits the quantum nature of light and is performed by using entangled photon pairs. The reconstruction of an image employs an iterative algorithm based on probabilistic mathematics. Later single-pixel imaging techniques that use a classical light source to exploit Helmholtz reciprocity [3] have been proposed. These techniques include GI [4] , [5] , [6] , [7] , computational imaging [8] , [9] , [10] , [11] and dual photography [1] , [12] , [13] . These single-pixel techniques can potentially capture a scene with indirect measurement where detectors sample the indirect light only. In other words, the detection unit needs not a direct line of sight to the imaged object. To achieve this, the key point is to increase the SNR in measurement. Several approaches aiming at increasing the SNR have been proposed, such as differential measurement [6] , [10] , [11] , illumination pattern normalization [7] , [10] , [11] , frequency-locked measurement [10] , [11] and so on. However, to our knowledge, no single-pixel technique can successfully achieve high-quality imaging with indirect measurement so far. In this paper, we report a single-pixel imaging technique that can reconstruct high-quality images by acquiring their Fourier spectrum. From the perspective of its physics nature, the technique is subject to the Helmholtz reciprocity. It allows indirect measurements in which a single-pixel detector capture a scene without directly looking at it. Thus, the detector can be placed wherever it can collect light signals from the scene, which is like a radio set that can be placed wherever it can receive the radio waves emitted by a station. The proposed technique employs the use of greyscale, analytic, harmonic sinusoid patterns (the real part of Fourier transform basis), instead of random speckle or binary basis patterns, for illumination. There are approaches to super-resolution microscopy with the use of the sinusoid structured illumination [14] , [15] , [16] . The proposed technique acquires the Fourier spectrum of the scene image with the four-step phase-shifting sinusoid illuminations. The desired image can be perfectly reconstructed by applying the two-dimensional (2D) inverse fast Fourier transform (IFT) algorithm. The phase-shifting illumination approach brings the elimination of noise that is statically the same. Particularly, when the sampling rate is far higher or lower than the flashing rate of the environmental light sources, the approach would largely cancel out the noise from the environmental illumination. Moreover, the sinusoid patterns are naturally normalized in intensity. Consequently each measurement collects half of the total flux on average, which not only benefits the efficiency of the illumination source’s available energy flux, but also ensures the detector is able to operate in the linear region with sufficient input light energy. In addition, the sinusoid patterns can be generated by several means. For example, a commercial digital projector displays the patterns in 24-bit mode; a programmable digital micromirror device (DMD) that displays the patterns in binary mode, and the defocusing [17] or the spatial filtering approach [16] is employed to make the resulting patterns sinusoidal; two coherent plane waves intersect at an angle to form a sinusoid pattern. What is more, the technique presented here is a compressive sampling [4] , [8] , [9] , [10] , [12] , [13] like approach. It applies measurement in the Fourier domain, where most natural images are sparse. More importantly, it is known that the large coefficients are concentrated at the low-frequency region of the Fourier domain. Thus, the technique is capable of reducing the number of measurements. In summary, the proposed technique has advantages of high SNR in indirect measurement and applicability in the real world. Experimental setup The schematic diagram of the proposed technique is shown in Fig. 1 . The scene consisted of a toy and an enlarged 1951 USAF resolution test pattern printed on a piece of A4 white paper. The test pattern had a number of features designed to allow for assessment of the image quality. The four-step phase-shifting sinusoidal patterns of different spatial frequency with 245 × 245 pixels were generated by the computer. The illumination patterns were of 256 greyscale levels and successively projected by a commercial digital projector. The illuminated area was 0.16 × 0.16 m 2 in size. We used two single-pixel detection units to collect the resulting light separately. Each unit was lensless and not able to directly observe the imaged scene. The projector switched the illumination patterns every 0.15 s and the detectors sampled synchronically. The scheme of the technique is also illustrated in Supplementary Movie 1 . 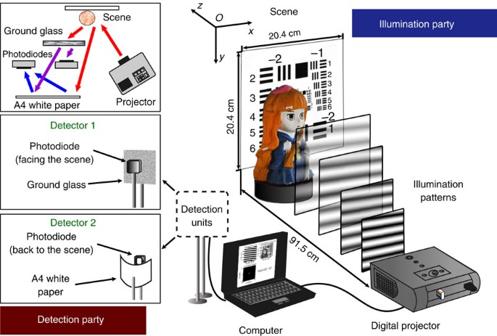Figure 1: Experimental setup. The digital projector (TOSHIBA Tp-95) illuminated the scene with the four-step phase-shifting sinusoidal structured light patterns. The detection unit (a photodiode, Hamamatsu S1227-1010BR, driven by an amplification circuit) collected the scattered reflected light from the scene and fed the resulting signals to the computer for a computational reconstruction of images. We used two different detection units for image reconstructions, which were a photodiode covered with a piece of ground glass (detector 1) and a reversely placed photodiode with a piece of A4 white paper as a reflecting diffuser (detector 2). The optical path is on the left top. Figure 1: Experimental setup. The digital projector (TOSHIBA Tp-95) illuminated the scene with the four-step phase-shifting sinusoidal structured light patterns. The detection unit (a photodiode, Hamamatsu S1227-1010BR, driven by an amplification circuit) collected the scattered reflected light from the scene and fed the resulting signals to the computer for a computational reconstruction of images. We used two different detection units for image reconstructions, which were a photodiode covered with a piece of ground glass (detector 1) and a reversely placed photodiode with a piece of A4 white paper as a reflecting diffuser (detector 2). The optical path is on the left top. Full size image Imaging in absence of environmental illumination Our first goal was to reconstruct a 2D image (245 × 245 pixels) of the 3-D scene by using a lensless single-pixel detector without direct observation. Note that there are no illumination sources except the projector in this case. A commercial digital projector was used to illuminate the scene. As Fig. 1 shows, detector 1, whose photosensitive surface facing the scene, was covered with a piece of ground glass with a thickness of 5.1 mm. A part of the light reflected from the surface of the objects in the scene passed through the glass and became partly scattered. Thus, the light that detector 1 collected was a mixture of direct and indirect light. Detector 2 was reversely placed, with its photosensitive surface back to the scene. A piece of A4 white paper was used as a reflecting diffuser. Detector 2 collected the light scattered by the diffuser. Thus, the light that detector 2 collected could be viewed as only indirect light. To perfectly reconstruct a 245 × 245-pixel image, the same number of Fourier coefficients is required. We used the four-step phase-shifting sinusoid illumination for Fourier spectrum acquisition. Each Fourier coefficient was obtained with four measurements. As the Fourier spectrum of a real-valued signal is conjugate symmetric, half of the coefficients are redundant. Thus, in our case, the number of measurements for the Fourier spectrum with a coverage of 100% is 120052. It took over 5 h to obtain a full-resolution complete frame. Reconstructed images from detectors 1 and 2 with a spectrum coverage from 1% to 100% are given in Fig. 2 . As the figure shows, the proposed technique can achieve clear images by collecting either a mixture of direct and indirect light or only indirect light. When the number of measurements is in common, the images from detector 2 appear slightly noisy than those from detector 1. It is because the light that detector 2 collected was relatively weak, which results in a lower SNR. 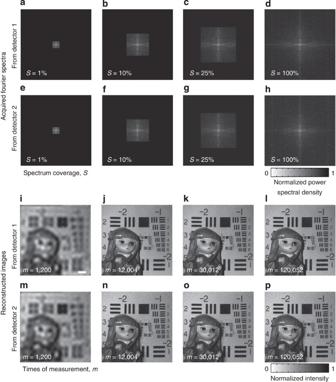Figure 2: Acquired Fourier spectra from detectors 1 and 2 with spectrum coverage from 1 to 100% and corresponding reconstructed images. (a–d) are the density distributions of Fourier spectrum acquired from detector 1, whereas (e–h) from detector 2. (i–l) are the reconstructed images corresponding to (a–d) and (m–p) correspond to (e–h), respectively. Note that we show the absolute value of the Fourier spectrum on a logarithm scale to render them visible. The images are reconstructed by using the 2D discrete IFT algorithm. No post processing has been applied to the reconstructed images. Scale bar, 2 cm. Figure 2: Acquired Fourier spectra from detectors 1 and 2 with spectrum coverage from 1 to 100% and corresponding reconstructed images. ( a – d ) are the density distributions of Fourier spectrum acquired from detector 1, whereas ( e – h ) from detector 2. ( i – l ) are the reconstructed images corresponding to ( a – d ) and ( m – p ) correspond to ( e – h ), respectively. Note that we show the absolute value of the Fourier spectrum on a logarithm scale to render them visible. The images are reconstructed by using the 2D discrete IFT algorithm. No post processing has been applied to the reconstructed images. Scale bar, 2 cm. Full size image The proposed technique is a compressive sampling like approach. In general, most information of a natural scene concentrates on low-frequency components. With the strategy that the Fourier spectrum acquired in the order from lower to higher frequencies, the quality of the reconstructed images improves with a rapid convergence. The scene can be roughly recognized from the images with only 1% of spectrum coverage. When spectrum coverage reaches 10%, the quality remarkably improves. The differences among the images reconstructed from a spectra with a coverage from 25% (half of Nyquist measurements) to 100% (double of Nyquist measurements) are nearly unnoticeable. Since natural images are sparse in the Fourier domain, the Fourier spectrum measurement can reconstruct faithful-quality images by performing the sub-Nyquist measurements. Helmholtz reciprocity permits the roles interchanged between an illumination source and a detection unit. Therefore, the field of view of the reconstructed images is determined by the position of the projector to the scene, while the location of the shades profile is set by the position of the single-pixel detector. The proposed technique performs Fourier spectrum measurements to obtain the desired image. Random noise in measurement would equally affect each frequency component in the spectrum. As a result, the primary noise for the proposed technique should be the white noise that is characterized by a constant power spectral density. Increasing the exposure time of the detector is an effective approach to reduce the white noise, which achieves a temporal average. In addition, there exists a periodic noise in the originally reconstructed images in our experiments. The noise is caused by the discretization introduced by the digital projector that operates in the 24-bit mode. The illumination patterns are digitalized by the digital projector, which leads to several Fourier coefficients with unusually larger modulus than their neighbours in the spectrum. Fortunately, the locations of these Fourier coefficients are of regularity so that they can be picked out with a common spectral mask and reasonably replaced by their neighbour mean. 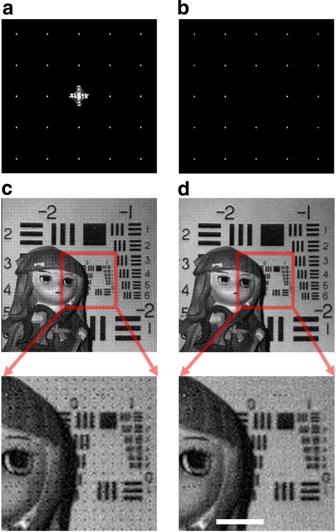Figure 3: Illustration of periodic noise reduction. By applying thresholding to the discrete 2D Fourier spectrum (modulus) image acquired from detector 1, it yields (a) where the white pixels represent coefficients with greater modulus than the threshold. (b) Is the spectral mask that isolates the false coefficients for further correction. The generation of the mask is depicted inSupplementary Methodsin detail. (c) and (d) Are the reconstructed images with their partial enlargement before and after periodic noise reduction process, respectively. Comparingcwithd, the visible periodic noise resulted from the discretization of the digital projector has been effectively eliminated. Scale bar, 2 cm. Figure 3 briefly illustrates the process of periodic noise reduction by frequency domain filtering and a detailed illustration is given in Supplementary Methods . The periodic noise could be avoided by using other aforementioned sinusoid pattern generation methods. Figure 3: Illustration of periodic noise reduction. By applying thresholding to the discrete 2D Fourier spectrum (modulus) image acquired from detector 1, it yields ( a ) where the white pixels represent coefficients with greater modulus than the threshold. ( b ) Is the spectral mask that isolates the false coefficients for further correction. The generation of the mask is depicted in Supplementary Methods in detail. ( c ) and ( d ) Are the reconstructed images with their partial enlargement before and after periodic noise reduction process, respectively. Comparing c with d , the visible periodic noise resulted from the discretization of the digital projector has been effectively eliminated. Scale bar, 2 cm. Full size image Imaging in presence of environmental illumination Environmental illumination is challenging for the existing single-pixel imaging techniques. Our second goal was to demonstrate the technique’s ability to eliminate the background noise. We introduced an environmental illumination with fluorescent lamps flashing at a rate of 100 Hz. The environmental illumination contributes to the noise that reduces the SNR. 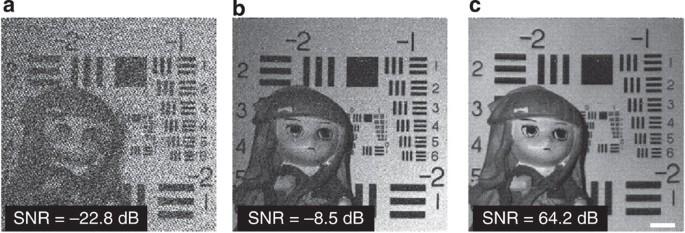Figure 4: Images with different SNRs. The images are reconstructed from (a) detector 2 with environmental illumination of fluorescent lamps, (b) detector 1 with environmental illumination of fluorescent lamps and (c) detector 1 without any environmental illumination, respectively. The SNRs are computed according to the equation (S9). Periodic noise reduction has been applied. Scale bar, 2 cm. Figure 4 shows the images reconstructed from the different SNRs. The proposed technique is capable of reconstructing clear images even from a negative SNR with the employment of phase-shifting illuminations that cancel out the background noise efficiently. Such a property makes the proposed technique practical in use. The SNR calculations are given in Supplementary Methods . Figure 4: Images with different SNRs. The images are reconstructed from ( a ) detector 2 with environmental illumination of fluorescent lamps, ( b ) detector 1 with environmental illumination of fluorescent lamps and ( c ) detector 1 without any environmental illumination, respectively. The SNRs are computed according to the equation (S9). Periodic noise reduction has been applied. Scale bar, 2 cm. Full size image The proposed technique employs the use of sinusoid patterns for structured illumination. It performs Fourier spectrum measurements to acquire the image information. The illumination patterns are deterministically represented in mathematics and can be generated by a few methods. The orthogonality of the patterns allows the desired image to be perfectly reproduced with a fixed and finite number of measurements in the absence of noise. The number is equal to that of the total pixels on the final image. Moreover, natural images can be sparsely represented in the Fourier domain. To increase the SNR, the four-step phase-shifting sinusoid pattern illumination is employed for differential measurements. The four-step phase-shifting sinusoid illumination can remove the direct current (DC) component but doubles the number of measurement. Although one might use other orthogonal pattern sets to achieve the features depicted above, the phase-shifting sinusoid patterns set has its additional feasibilities including: (1) Various methods are available for pattern generation. For instance, the sinusoid patterns can be generated by the interference of two coherent plane waves. It should be noted that the greyscale sinusoid patterns can also be generated by the use of a programmable DMD operating in binary mode. The resulting binary (stripe) patterns can be converted to greyscale (fringe) by employing the defocusing techniques or the spatial low-pass filtering. DMDs with binary projection rates of 22 kHz and above are becoming common, which allows up to kilo-per-second measurements. (2) The N -step phase-shifting sinusoid illuminations ( N ≥3) is able to assemble the Fourier spectrum of the image and eliminate the DC term in measurements. The more the steps of phase shifts involved, the longer the measurement time will be. (3) Rapid convergence of image quality in reconstruction is observed. Since natural images are generally sparse in the Fourier domain (for example, most information concentrates in the low-frequency region), the proposed technique obtains the Fourier spectrum with an increasing spatial frequency (from low to high) allowing the reconstruction of a recognizable image with a small number of measurements. (4) Self-error correction can be achieved. As it is carried out in the frequency domain, the proposed technique can be assisted with the existing well-developed frequency-domain processing algorithms for image enhancements. Incorrect measurements due to noise could be identified and even corrected. (5) The proposed technique offers fast computation along with a small memory requirement. The image reconstruction process employs 2D IFT algorithm, which has a fast implementation. The illumination patterns are predetermined and need not be stored on a computer. We have noted that there exist some possible factors contributing to the additive noise on reconstructed images: discretization of illumination patterns (quantization of greyscale and position), nonlinear responses of the photodiode, circuit noise at the amplifier and the photodiode. The noticeable ‘grid’ on the images in our experiment is introduced by the discretization of the illumination pattern. The quantization of the patterns’ greyscale levels would violate the normalization of the image intensity in the case of some spatial frequencies. The reduction for such periodic noise is introduced in detail in Supplementary Methods . The quality of the reconstructed images can be further improved by increasing the contrast of the illumination patterns and the SNR of detectors. For full-colour imaging, one can use three photodiodes covered with spectral filters to reconstruct the red, green and blue sub-images. We have experimentally validated this approach. The scheme and the results are presented in Supplementary Fig. 5 . However, the proposed technique has two limitations. One is that it requires an illumination source with spatial resolution in a direct line of sight of the imaged objects, although the detectors need not observe the objects directly. The other is that it can only be used in static measurement so far. In conclusion, this paper introduces a single-pixel imaging technique capable of reconstructing images from indirect measurements in which a single-pixel detector does not need to directly observe the imaged objects. The indirect measurements lead to a feasible placement of the detector. The technique can still work even under environmental illumination. The technique acquires the Fourier spectrum of the desired image with the use of a four-step phase-shifting sinusoid illumination. Moreover, the proposed technique can reproduce a clear image of a natural scene from sub-Nyquist samples. In terms of computational efficiency, the image reconstruction employs the use of 2D fast IFT algorithm rather than any iterative or minimization algorithms. The analytic Fourier mathematics that the proposed technique is based on enables perfect image reproductions in principle. Various approaches to illumination pattern generation bring feasibilities into practical uses. The technique can be extended to large field-of-view imaging in various wavebands. Principle of the proposed technique The proposed single-pixel imaging technique is based on the theorem of Fourier transform. It obtains the Fourier spectrum of a scene image by illuminating the scene with phase-shifting sinusoidal structured light patterns and using a detector, which has no spatial resolution, to collect the resulting light. In our experiment, the four-step phase-shifting sinusoid illumination was employed for the spectrum acquisition. As we demonstrate below, the phase-shifting approach can not only assemble the desired Fourier coefficients, but also effectively eliminate errors that are statically the same. High SNR can therefore be obtained, which makes the proposed technique able to work with the sampled indirect light. The final image is reconstructed by applying the fast IFT algorithm to the Fourier spectrum acquired. The Fourier transform provides a perspective that an image consists of a weighted sum of harmonic 2D structured light patterns with different frequencies, as Supplementary Fig. 2 shows. Therefore, it is possible to reconstruct the image if the weight of each (that is, Fourier coefficient) corresponding frequency is known. Each weight can be obtained by four measurements, that is, to successively illuminate the scene with four sinusoid patterns with a phase shift of π / 2 . The illumination patterns are greyscale images instead of the commonly used binary ones. In addition, the patterns have the same global intensity, which omits normalization. With the illumination P being known, the measurement process refers to the acquistion of the corresponding Fourier coefficient, C . The coefficients are complex numbers. As each complex number generally takes 16 b for storage, the proposed technique just occupies 2 Mb to store the data for a 512 × 512-pixel image. A 2D sinusoid pattern is specified with its spatial frequency ( f x , f y ) and initial phase, φ . It is given by: where ( x , y ) represents the 2D Cartesian coordinates in the scene, a is the DC term equal to the average image intensity and b represents the contrast. By illuminating a scene with a pattern, the total intensity of reflected light arising from the structured light source can be expressed as: where Ω represents the illuminated area, R is the distribution of the surface reflectivity of the imaged objects in the scene. The integration in equation (2) implies that the detectors can collect any kind of light for imaging, despite the light being a direct light, indirect light or a mixture of both. It is because the effective light signal is independent on the propagation path, as long as the media in the scene are linear and static. When a single-pixel detector is used, it can collect a part of the reflected light that reaches its photosensitive surface. Thus, the total response, D φ , can be expressed as: where k depends on the size and the location of the detector, D n represents the response of environmental illuminations. The four-step phase-shifting approach allows each complex Fourier coefficient C ( f x , f y ) to be obtained by four responses corresponding to the illumination patterns (that is, P 0 , P π /2 , P π and P 3 π /2 ). These four patterns are with the same spatial frequency ( f x , f y ), and a constant phase shift Δ ϕ = π /2 between two adjacent patterns. Applying the following equation can obtain the proportional Fourier spectrum of R and cancel out the DC term: where j denotes the imaginary unit and F the Fourier transform. Equation (4) is a differential measurement for which the DC term is removed efficiently. In other words, the noise caused by environmental illumination can be effectively eliminated. By applying the IFT to the right hand side of equation (4), it yields: where F −1 denotes the inverse Fourier transform operator. The result of the inverse transform is the final image whose gray values are proportional to the reflectivity R ( x , y ). A detailed deduction is provided in Supplementary Methods . How to cite this article : Zhang, Z. et al . Single-pixel imaging by means of Fourier spectrum acquisition. Nat. Commun. 6:6225 doi: 10.1038/ncomms7225 (2015).